In vivorecordings of brain activity using organic transistors In vivo electrophysiological recordings of neuronal circuits are necessary for diagnostic purposes and for brain-machine interfaces. Organic electronic devices constitute a promising candidate because of their mechanical flexibility and biocompatibility. Here we demonstrate the engineering of an organic electrochemical transistor embedded in an ultrathin organic film designed to record electrophysiological signals on the surface of the brain. The device, tested in vivo on epileptiform discharges, displayed superior signal-to-noise ratio due to local amplification compared with surface electrodes. The organic transistor was able to record on the surface low-amplitude brain activities, which were poorly resolved with surface electrodes. This study introduces a new class of biocompatible, highly flexible devices for recording brain activity with superior signal-to-noise ratio that hold great promise for medical applications. Most breakthroughs in our understanding of the basic mechanisms of information processing in the brain have been obtained by means of recordings from electrodes implanted into, or placed on the surface of the brain. Such recordings allowed the discovery of place cells, grid cells, mirror neurons [1] , [2] , [3] and more. They also provided an insight into the organization of the brain [4] , and showed that oscillations constitute the hallmark of brain activity. These oscillations are divided into different frequency bands, from ultraslow to ultrafast, including delta (0.5–3 Hz), theta (4–12 Hz), gamma (40–80 Hz), ripples (100–200 Hz) and sleep spindles (>500 ms long 10–14 Hz oscillations) [4] , [5] . Specific oscillations are also recorded in pathological contexts such as spike and wave discharges (SWDs) between 7 and 11 Hz in experimental models of absence epilepsy. For other types of epilepsies, the epileptogenic regions may be determined by assessing the presence of interictal spikes and/or very fast ripples (>200 Hz) [6] . State-of-the-art recordings are currently performed with microfabricated arrays of metal electrodes (silicon probes, Utah arrays and tetrodes [7] ), which capture the local field potentials (LFPs) generated by the spatio-temporal summation of current sources and sinks (caused by the flux of ions through ion channels localized in the cell membrane) in a given brain volume [4] . Such probes are also being used in the clinic to improve diagnosis and treatments. For example, stereoelectroencephalography and electrocorticography (ECoG) probes are used to localize epileptogenic zones and to provide functional mapping of the brain before surgery [8] , [9] , [10] , [11] , [12] . Although ECoG probes are easier to use than stereoelectroencephalography probes, recordings performed on the brain surface pick up a highly integrated, global signal, which corresponds to the summation of different signals generated at different depths. Hence, ECoG probes are not able to accurately detect activities generated by smaller cell assemblies, except those generated right below an electrode. In addition to clinical applications, microfabricated probes are also likely to have a key role in the design of future brain-machine interfaces [13] , [14] . However, major technological advances are still needed; the probes must be fully biocompatible (to enable long-term recordings), small/thin (to decrease invasiveness), highly conformable (to comply with the complex three-dimensional architecture of the brain) and, most importantly, must provide an increased signal-to-noise ratio (SNR) through a built-in pre-amplification/processing system. Neurons and brain networks generate small electric potentials, which are difficult to extract from noise when recorded with classical electrodes made of metals such as Ir, Pt and Au. Advances in microelectronics have given rise to the electrolyte/oxide/silicon field-effect transistor (FET), a more sophisticated device that has been used to measure in vitro signals from cell cultures and tissues slices [15] , [16] , [17] , [18] . In these devices, the transmembrane current from a neuron in the electrolyte polarizes the gate dielectric and leads to a change in the conductance of the underlying silicon channel. The use of transistors rather than simple electrodes provides the potential of increased SNR due to local amplification endowed by the transistor circuit, and of massive integration, which is possible through the use of matrix-addressing technology developed for flat-panel displays [15] , [16] , [17] , [18] . These advances, however, have so far been limited to in vitro recordings, mostly because of the poor biocompatibility of the oxide layer of the FETs. Although silicon FETs have recently been integrated into in vivo probes as a means of enabling simultaneous addressing of hundreds of electrodes [19] , the recordings were carried out by classical electrodes, whereas the transistors themselves were carefully encapsulated to avoid direct contact with the brain. An alternative transistor architecture, termed the organic electrochemical transistor (OECT), was developed in the ‘80s (ref. 20 ). In contrast to FETs, where an oxide separates the channel from the electrolyte and prohibits any ion transport between these two layers, the channel of OECTs is in direct contact with an electrolyte. As a result, the channel/electrolyte interface constitutes an integral part of the operation mechanism of OECTs. State-of-the-art OECTs are based on the conducting polymer poly(3,4-ethylenedioxythiophene) doped with polystyrene sulfonate (PEDOT:PSS) [21] . This material is a heavily doped p- type organic semiconductor, in which holes on the PEDOT chains (the semiconductor) are compensated by sulfonate anions on the PSS (the dopant) [22] . The application of a positive bias on a gate electrode immersed in the electrolyte causes cation injection into the PEDOT:PSS film. These cations compensate the sulfonate anions and dedope the PEDOT, thereby decreasing the drained current [23] . PEDOT:PSS OECTs work, therefore, in the depletion mode. Accumulation-mode OECTs, based on intrinsic organic semiconductors, have also been reported, but they typically show higher operation voltages [24] . As OECTs capture ion fluxes [25] , [26] , they constitute the optimal solution to measure electrophysiological signals—fluctuations of the electric field (field potentials), generated by the movement of ions [27] . OECTs offer additional advantages that make them attractive candidates for neural interfacing, including cytocompatibility and straightforward integration with mechanically flexible (hence conformable) substrates [17] , [18] . Here we demonstrate the first in vivo use of a transistor to record brain activity. We fabricated highly conformable arrays of OECTs and used them to carry out ECoG on the somatosensory cortex of rats. Simultaneous recordings from penetrating and surface electrodes were used to validate the transistor recordings in two animal models. Compared with surface electrodes, OECTs showed a superior SNR due to local amplification. They also revealed a richer electrophysiological signal, similar to that obtained with penetrating electrodes. Structure of the transistor arrays We fabricated ECoG probes that contained OECTs, as well as electrodes made from PEDOT:PSS. Micrographs of an ECoG probe and the layouts of a transistor and an electrode are shown in Fig. 1 . A 2-μm thick parylene film was used as the substrate, onto which Au and PEDOT:PSS films were photolithographically patterned. Au served as source and drain electrodes, electrode pads and interconnect lines, whereas PEDOT:PSS was used for the transistor channel and the surface electrodes. A second 2-μm thick parylene film, appropriately patterned to allow access to the channel and to the electrodes, was deposited on top and used as the insulator ( Fig. 1c ). The total thickness of the arrays was ~4 μm, resulting in probes that were highly conformable yet had enough mechanical strength to be self-supporting and allow manipulation during surgery. Each probe contained 17 transistors with a channel length of 6 μm and a channel width of 15 μm, and 8 electrodes with dimensions of 12 × 12 μm 2 . The Au structures were completely covered with PEDOT:PSS or parylene, and were not exposed to the electrolyte. Parylene is a Food and Drug Administration-approved polymer used in implantable devices, such as pacemakers, whereas PEDOT-based electrodes have been extensively used as recording electrodes in vivo [28] , and have been shown to outperform traditional metal electrodes in chronic experiments [29] . Implanted in the brain, both parylene and PEDOT:PSS elicit a very small glial response ( Supplementary Fig. S1 ). Therefore, the arrays exposed biocompatible-only materials to the brain. A through hole at the centre of the array allowed the insertion of a silicon probe. At the other end of the probe, pads compatible with a zero insertion force connector allowed easy interfacing to electronics for recording, as shown in the inset of Fig. 1a . 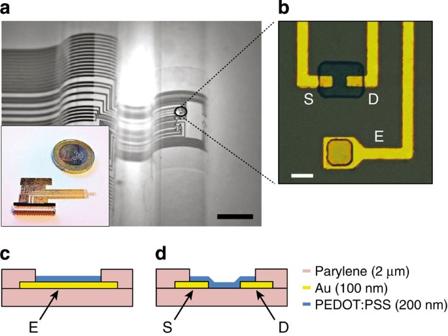Figure 1: Structure of the ECoG probe. (a) Optical micrograph of the probe conforming onto a curvilinear surface. Scale bar, 1 mm. The inset shows an image of the whole probe, in which the transistor/electrode arrays are on the right-hand side, whereas the external connections, onto which a zero insertion force (ZIF) connector is attached, are on the left-hand side. (b) Optical micrograph of the channel of a transistor and a surface electrode, in which the Au films that act as source (S), drain (D) and electrode pad (E) are identified. Scale bar, 10 μm. (c,d) Layouts of the surface electrode and of the transistor channel, respectively (not to scale). Figure 1: Structure of the ECoG probe. ( a ) Optical micrograph of the probe conforming onto a curvilinear surface. Scale bar, 1 mm. The inset shows an image of the whole probe, in which the transistor/electrode arrays are on the right-hand side, whereas the external connections, onto which a zero insertion force (ZIF) connector is attached, are on the left-hand side. ( b ) Optical micrograph of the channel of a transistor and a surface electrode, in which the Au films that act as source (S), drain (D) and electrode pad (E) are identified. Scale bar, 10 μm. ( c , d ) Layouts of the surface electrode and of the transistor channel, respectively (not to scale). Full size image In vitro characterization The transistors were characterized in vitro using Ringer’s solution as the electrolyte and a stainless-steel gate electrode. Their output characteristics, shown in Fig. 2a for a drain voltage ( V D ) between 0 and −0.5 V and a gate voltage ( V G ) between 0 and 0.5 V, are typical for operation in the depletion regime [23] . Upon application of a positive gate voltage, cations from the electrolyte enter the polymer film and dedope it, decreasing the drain current ( I D ). Owing to the absence of a gate oxide and to the high conductivity of PEDOT:PSS, the transistors show a low-operation voltage, which permits operation in aqueous environments. The corresponding transfer curve for V D =−0.4 V, shown in Fig. 2b , exhibits a slope that increases with gate voltage. This is reflected in a transconductance that increases with V G up to 0.42 V, where it reaches a maximum of 900 μS. Normalized for channel width, this value (60 × 10 3 μS mm −1 ) is two orders of magnitude larger than that of planar silicon-based FETs used in in vitro neural interfaces [16] and three orders of magnitude larger than that of typical organic FETs [30] , which reflects the efficient gating of the polymer channel due to direct contact with the electrolyte. The transconductance was constant up to 1 kHz ( Supplementary Fig. S2 ), which is above the fastest oscillations recorded in the brain [31] . It should be noted that the steady-state gate current was less than 10 nA for V D =−0.4 V and V G =0.5 V. Device statistics and stability data are shown in Supplementary Figs S3–S5 . 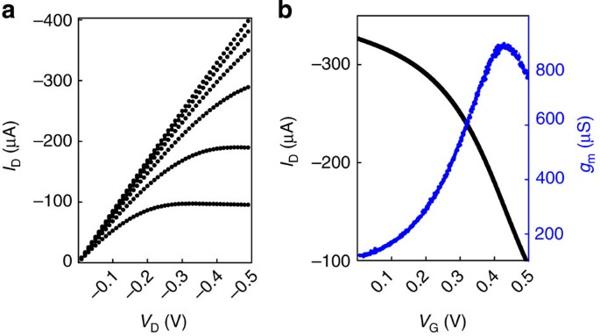Figure 2:In vitrocharacterization of the transistor. (a) Output characteristics showing the drain current,IDas a function of drain voltage,VDfor a gate voltage,VGvarying from 0 V to 0.5 V (with a step of 0.1 V) of a PEDOT:PSS transistor in Ringer’s solution and with a stainless-steel gate electrode. (b) Transfer curve and resulting transconductance atVD=−0.4 V. Figure 2: In vitro characterization of the transistor. ( a ) Output characteristics showing the drain current, I D as a function of drain voltage, V D for a gate voltage, V G varying from 0 V to 0.5 V (with a step of 0.1 V) of a PEDOT:PSS transistor in Ringer’s solution and with a stainless-steel gate electrode. ( b ) Transfer curve and resulting transconductance at V D =−0.4 V. Full size image In vivo characterization As the first application of OECT-based ECoGs is likely to be for epilepsy diagnosis and cortical mapping, we first characterized the in vivo performance of the transistors in an experimental model of epileptiform activity in rats. Animals were deeply anaesthetized and a craniotomy was performed. The ECoG probe was placed on the somatosensory cortex, and a silicon probe displaying a linear array of Ir electrodes was implanted through the hole in the centre of the ECoG probe ( Fig. 3a ). The transistor was wired in a common source configuration ( Fig. 3b ), with the grounded screw used as the gate electrode. We used V D =−0.4 V and V G =0.3 V. Bicuculline, a GABA A receptor antagonist, was perfused on the surface of the brain. Blockade of GABAergic inhibition invariably leads to the genesis of spikes that resemble interictal spikes [32] . Representative recordings from an OECT, a PEDOT:PSS surface electrode, and the penetrating electrodes of the silicon probe are shown in Fig. 3c . The temporal coincidence of the peaks in the data indicates that the transistor records the same information as the electrodes. The background activity signal is shown at the same scale for the three recording devices, demonstrating the far superior SNR of the transistor. The SNR was calculated by taking the highest peak during a period of epileptiform activity and the standard deviation (STD) of the background during a period of low biological activity. For the OECT recordings, these values were 1.5 μA and 9.5 nA, respectively, yielding an SNR of 44 dB, whereas the PEDOT:PSS surface electrode yielded an SNR of 24.2 dB (4.3 mV peak, 0.26 mV STD background). Although the OECT and the surface electrode were next to one another, and thus picked up the same activity in terms of fluxes of charges on the surface of the brain, the transistor recorded with a much higher SNR. The biological origin of this signal was confirmed by performing current source density (CSD) analysis on the silicon probe recordings ( Fig. 3d ). The latter reveals the presence of the source and sink (hence, the dipole) generating the epileptiform spike. It should be noted that all recordings were bandpass filtered between 0.1 and 200 Hz (see Methods), to minimize the influence of the acquisition system on the SNR. Although this does not completely eliminate the influence of the acquisition system, it still demonstrates the superior gain provided by the local amplification of the signal by the transistor circuit of Fig. 3b . 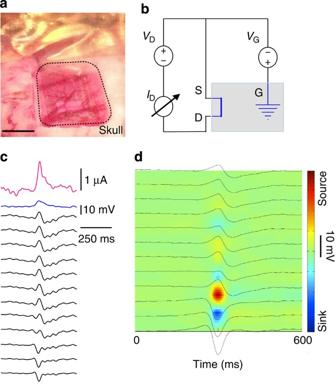Figure 3: Validation in Wistar rats. (a) Optical micrograph of the ECoG probe placed over the somatosensory cortex, with the craniotomy surrounded by dashed lines. Scale bar, 1 mm. (b) Wiring layout of the transistor, with the blue box indicating the brain of the animal. (c) Recording of a bicuculline-induced epileptiform spike from a transistor (pink), a PEDOT:PSS surface electrode (blue) and 12 of the 16 Ir-penetrating electrodes (black). The transistor was biased withVD=−0.4 V andVG=0.3 V, and the scale of 10 mV is for both surface and penetrating electrodes. (d) Current source density map of a bicuculline-induced epileptiform spike (44 events averaged shown as an overlay) showing a strong sink and source around the reversal of the event, in the deeper layers of the somatosensory cortex. Figure 3: Validation in Wistar rats. ( a ) Optical micrograph of the ECoG probe placed over the somatosensory cortex, with the craniotomy surrounded by dashed lines. Scale bar, 1 mm. ( b ) Wiring layout of the transistor, with the blue box indicating the brain of the animal. ( c ) Recording of a bicuculline-induced epileptiform spike from a transistor (pink), a PEDOT:PSS surface electrode (blue) and 12 of the 16 Ir-penetrating electrodes (black). The transistor was biased with V D =−0.4 V and V G =0.3 V, and the scale of 10 mV is for both surface and penetrating electrodes. ( d ) Current source density map of a bicuculline-induced epileptiform spike (44 events averaged shown as an overlay) showing a strong sink and source around the reversal of the event, in the deeper layers of the somatosensory cortex. Full size image In the above experiments, the evaluation of the OECT performance was obtained by triggering epileptiform activity with bicuculline. In a second set of experiments, we used a more relevant experimental model, the Genetic Absence Epilepsy Rat from Strasbourg (GAERS) [33] . This model has been validated in terms of isomorphism, homology and pharmacological predictability to be reminiscent of typical absence epilepsy, a form of generalized non-convulsive epilepsy. GAERS rats show spontaneous large amplitude SWDs at a frequency between 7 and 11 Hz, associated with behavioural arrest and slight perioral automatisms. Despite the fact that deep anaesthesia alters the expression of SWDs in GAERS rats, pathological epileptiform activity could be recorded ( Fig. 4a ) from the OECT, the PEDOT:PSS surface electrode and from Ir-penetrating electrodes of a silicon probe implanted in the first three superficial layers of the somatosensory cortex. The transistor is shown again to outperform the surface electrode: the SNR for the OECT was 52.7 dB (1.3 μA peak, 3 nA STD background), and 30.2 dB (13 mV peak, 0.4 mV STD background) for the PEDOT:PSS surface electrode. For the sake of completeness, the SNR for the Ir-penetrating electrode was 32.0 dB (10 mV peak, 0.3 mV STD background), although the different location of the probe (depth versus surface recording) does not permit a direct comparison. 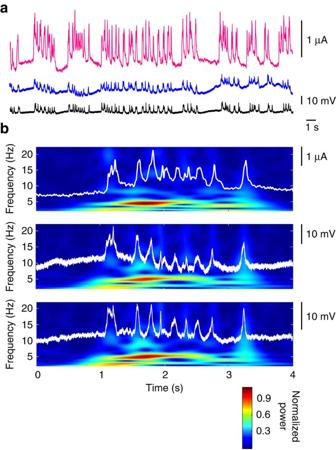Figure 4: Validation in GAERS rats. (a) Recordings from an OECT (pink), a PEDOT:PSS surface electrode (blue) and an Ir-penetrating electrode (black). The transistor was biased withVD=−0.4 V andVG=0.3 V, and the scale of 10 mV is for both surface and penetrating electrodes. Note the superior SNR of the OECT as compared with the surface electrode. (b) Time–frequency analysis of epileptiform activity during a short period, recorded by an OECT (top), a PEDOT:PSS surface electrode (middle) and an Ir-penetrating electrode (bottom). Figure 4: Validation in GAERS rats. ( a ) Recordings from an OECT (pink), a PEDOT:PSS surface electrode (blue) and an Ir-penetrating electrode (black). The transistor was biased with V D =−0.4 V and V G =0.3 V, and the scale of 10 mV is for both surface and penetrating electrodes. Note the superior SNR of the OECT as compared with the surface electrode. ( b ) Time–frequency analysis of epileptiform activity during a short period, recorded by an OECT (top), a PEDOT:PSS surface electrode (middle) and an Ir-penetrating electrode (bottom). Full size image The time–frequency analysis of epileptiform activity during a short period revealed the presence of typical oscillations around 5Hz ( Fig. 4b ). Moreover, for better illustration of the SNR improvement the corresponding time traces were normalized according to the peaks of the activity. Electrodes and OECTs alike detected the same signal, in keeping with the fact that SWDs are generalized discharges, which sum up to give rise to a strong signal on the surface. The situation was, however, remarkably different during recordings in between epileptiform activities, where low-amplitude oscillations in the 4–14 Hz frequency range were observed. Time–frequency analysis of recordings showed that the OECT and the Ir-penetrating electrode were able to pick up these low-amplitude signals, whereas the PEDOT:PSS surface electrode showed poor resolution ( Fig. 5 ). The SNR was 22.3 dB for the OECT (300 nA peak, 23 nA STD background), 13.5 dB for the surface electrode (3.5 mV peak, 0.74 mV STD background) and 18.2 dB for the penetrating electrode (3 mV peak, 0.37 mV STD background), with the caveat that the latter recorded in a different location. It should be noted that the depth of anaesthesia used here prevented us from assessing the presence of faster oscillations (such as gamma oscillations) in this case. 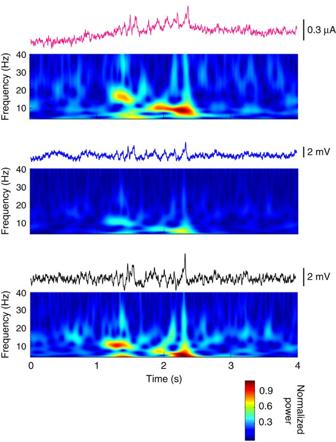Figure 5: Recordings of low-amplitude oscillations. Recordings from an OECT (top), a PEDOT:PSS surface electrode (middle) and an Ir-penetrating electrode (bottom), shown together with their corresponding time–frequency analysis plots (normalized TF energy), scaled to their minimum/maximum values. These oscillations, which have a lower amplitude than SWD, are picked up equally well by the OECT and the Ir-penetrating electrode, but are not well-resolved by the PEDOT:PSS surface electrode. Figure 5: Recordings of low-amplitude oscillations. Recordings from an OECT (top), a PEDOT:PSS surface electrode (middle) and an Ir-penetrating electrode (bottom), shown together with their corresponding time–frequency analysis plots (normalized TF energy), scaled to their minimum/maximum values. These oscillations, which have a lower amplitude than SWD, are picked up equally well by the OECT and the Ir-penetrating electrode, but are not well-resolved by the PEDOT:PSS surface electrode. Full size image The temporal coincidence of the OECT and electrode recordings confirms that both devices record LFPs. The key difference between a transistor and an electrode, however, lies in the fact that the former is an active device, which, when biased as shown in Fig. 3b , forms a circuit that acts as a voltage-controlled current-source amplifier. A voltage-controlled current-source amplifier transforms voltage modulations at the input loop (gate) to current modulations at the output loop (drain), while amplifying the signal power at the same time. For the case of V D =−0.4 V and V G =+0.3 V used in the in vivo measurements, a small oscillation of 50 mV at gate results in an output current oscillation of 37 μA, as defined by the transconductance. At low frequencies, the resistive component dominates the input impedance of the OECT circuit; hence, the input current is determined by the DC bias and is smaller than 10 nA. Therefore, the input signal power is lower than 0.5 nW (=50 mV × 10 nA), whereas the output signal power is 15 μW (=0.4 V × 37 μA). In contrast, conventional electrode recordings are pre-amplified outside the head of the animal. This means that the leads and connections pick up noise that is pre-amplified as well, thereby decreasing the SNR. In general, a higher SNR translates into a shorter overall recording time to obtain the same information. For example, when recording evoked potentials it is necessary to average many individual signals. It also means that new, previously unobserved features can be recorded. Electrodes placed on the surface of the brain record the LFPs associated with the summation of the electrical activity of neural networks, which can be located very far from the recording site. In contrast, penetrating electrodes provide more local, and thus more precise, information on the activity of small populations of neurons. We have previously reported that PEDOT:PSS ECoG electrodes show a better SNR than classical Au electrodes placed on the surface of the brain [34] . However, PEDOT:PSS electrodes showed less definition as compared with both OECTs and depth electrodes. The use of OECTs for in vivo recordings thus constitutes a major breakthrough, as they are likely to record small and more local activities. This is particularly important in the field of epilepsy, where identifying zones generating high-frequency oscillations or microseizures is the key for diagnosis [6] , [35] . OECTs can also provide detailed information on local information processing when functional mapping of brain regions is performed in the operating room before surgery. The biocompatibility of OECTs and their highly conformable nature make them particularly suited for these applications. Small penetrating electrodes are used to capture single-unit recordings, which represent the activity of a single neuron located in the vicinity of the electrode [7] . This raises the question of whether an OECT placed on a penetrating probe will be able to record the single-unit activity, and what new information, if any, will be revealed by the higher SNR. These experiments are currently ongoing. Finally, OECTs can help answer basic questions in neuroscience about the coupling between electrical activity and metabolism. To function, the brain needs energy in the form of glucose, which is carried in the blood. A dysfunction in this supply system results in pathological activities. Hypometabolism, for example, is one signature of epileptic regions [36] . The question of how the brain makes use of glucose in different contexts has never been addressed precisely, because it requires the simultaneous recording of neuronal activity and glucose level at the single neuron scale. PEDOT:PSS OECTs coupled with the redox enzyme glucose oxidase have been shown to make simple yet sensitive glucose sensors [37] . Their integration with electrodes that probe electrophysiology is rather straightforward. Such multi-modal probes would, for the first time, record electrophysiology and metabolism with high spatial resolution. The impact of such probes would be considerable and widespread, in basic physiology, pathology and even in the clinic to interpret metabolic imaging. Transistor fabrication and characterization The fabrication and in vivo validation of PEDOT:PSS electrodes [34] and the patterning of PEDOT:PSS OECTs [38] were discussed in previous publications. Here we used an adapted fabrication process that involved the deposition and patterning of parylene, Au and PEDOT:PSS films as follows: Parylene C was deposited using an SCS Labcoater 2 to a thickness of 2 μm (at which thickness parylene films are pinhole-free). These films were patterned with the aid of a 4.6-μm thick layer of AZ9260 (MicroChemicals) photoresist and reactive-ion etching by an O 2 plasma (160 W, 50 sccm O 2 , 15 min) using an Oxford 80 plus. Metal pads and interconnects were patterned by a lift-off process. A photoresist, S1813 (Shipley), was spin-coated on the parylene film at 3,500 r.p.m., baked at 110 °C for 60 s, exposed to UV light (150 mJ cm −2 ) using a SUSS MJB4 contact aligner, and then developed using MF-26 developer. This was followed by the deposition of 5 nm of titanium and 100 nm of gold using a metal evaporator (Alliance Concept EVA450). Lift-off was performed using 1165 stripper. For the preparation of the PEDOT:PSS films, 20 ml of aqueous dispersion (PH-1000 from H.C. Stark) was mixed with 5 ml of ethylene glycol, 50 μl of dodecyl benzene sulfonic acid and 1 wt% of 3-glycidoxypropyltrimethoxysilane (as a cross-linker), and the resulting dispersion was spin-coated at 650 r.p.m. The films were subsequently baked at 140 °C for 1 h and were immersed in deionized water to remove any excess low-molecular weight compounds. The transistors were characterized in vitro using Ringer’s solution (150 mM sodium, 3 mM potassium, 2 mM calcium, 1 mM magnesium and 10 HEPES/NaOH to adjust the pH to 7.2) as the electrolyte. A stainless-steel screw was immersed in the electrolyte and used as the gate electrode. This was the same type of screw that was used as a gate electrode in the in vivo experiments (see below). A Keithley 2612A dual SourceMeter was used to bias the transistor and record the drain and gate currents. The time delay between sourcing voltages and measuring currents was 100 ms, which was found to be long enough for reaching steady-state. In vivo evaluation All protocols have been approved by the Institutional Animal Care and Use Committee of INSERM. Four ECoG probes were tested, two with Wistar rats and two with GAERS rats. The Wistar rats were obtained from Charles River, MA, and the GAERS rats were obtained from Antoine Depaulis (Grenoble-Institut des Neurosciences, Grenoble, France). Upon receipt, they were maintained under controlled environmental conditions (23 °C, 12 h light/dark cycle). The GAERS rats (females, weight of 188 and 196 g, respectively) were initially anaesthetized with 5% isoflurane (Forene, Abbott, France) in 0.5 l min −1 O 2 and maintained under anaesthesia with 2% isoflurane. To record faster oscillations, the depth of the anaesthesia was decreased by reducing the amount of isoflurane to 1.5%. The Wistar rats (males, weight of 505 and 551 g, respectively) were anaesthetized with a ketamine/xylazine mixture (35 and 1 mg kg −1 , intramuscularly). Additional doses of ketamine/xylazine (7 and 0.3 mg kg −1 , intramuscularly) were given as needed. For surgery, the head of the rat was immobilized in a stereotaxic apparatus. The body temperature was monitored and kept constant at 37.5°C with a heating pad. Two miniature stainless-steel screws were driven into the skull above the cerebellum, and served as ground and reference electrodes, respectively. A 5 × 3 mm 2 craniotomy was performed in the right hemisphere above the somatosensory cortex (centred at −4 mm in the anterio-posterior axis and −2 mm in the medio-lateral axis, relative to Bregma). The dura mater was removed and the ECoG array was slowly lowered on the surface of the brain. The surface of the cortex was regularly rinsed with a 0.12 M phosphate buffer (33.76 g NaH 2 PO 4 –H 2 O, 7.72 g NaOH in 1 l bidistilled H 2 O, pH 7.4). The ECoG probe was accessed through a Molex zero insertion force connector with flat flexible cable to flexible printed circuitry configuration. 40 μl of a 100 μM bicuculline solution (Sigma-Aldrich) were deposited with a micropipette onto the brain surface of the Wistar rats after the dura mater was removed. The recordings ( Fig. 3c ) were taken after sufficient time (20 min) for the effects of bicuculline to diffuse through the cortical layers. In the Wistar rats, an implantable probe (Neuronexus A1 × 16–3 mm 100–177, with a single, 3-mm long shank containing a linear array of 16 electrodes of 177 μm 2 area each, spaced at 100 μm from each other) was inserted through the centre of the ECoG in the cortex to reach a final depth of 2 mm. In the GAERS rats, an implantable probe with small pitch between the electrodes (Neuronexus A1 × 8–3 mm 50–177, with a single, 3-mm long shank containing a linear array of eight electrodes of 177 μm 2 area each, spaced at 50 μm from each other) was inserted through the centre of the ECoG array in the cortex to reach a final depth of 1 mm. The penetrating probes were connected to a multi-channel Digital Lynx 10S system (Neuralynx) through a X1 HST headstage (Plexon). The signals were amplified (X1,000), bandpass filtered (0.1 Hz–5 kHz) and acquired continuously at 32 kHz on the 64-channel Neuralynx system (16-bit resolution). Signals from the ECoG PEDOT:PSS electrodes were also acquired by the same amplifier and under the same conditions. A Keithley 2612A dual SourceMeter was used to bias the transistor and record the drain and gate currents continuously at 0.3 kHz. Background levels of the recordings The PEDOT:PSS surface electrode recording in Fig. 3c was filtered at 0.1–200 Hz (plus a 50 Hz notch), and we obtain a background level of 0.26 mV. When we digitally filter this recording with a 1–50 Hz bandpass filter, we obtain a background level of 0.2 mV. The electrode recordings in Fig. 4a were filtered at 0.1–200 Hz (plus a 50 Hz notch), and we obtain background levels of 0.4 and 0.3 mV for the surface electrode and for the penetrating electrode, respectively. When we digitally filter the recordings with a 1–50 Hz bandpass filter, we obtain background levels of 0.2 and 0.1 mV for the surface electrode and for the penetrating electrode, respectively. Post-acquisition data treatment All recordings (from electrodes and OECTs alike) were digitally filtered with a 0.1–200 Hz bandpass filter to minimize the contribution of the frequency response of the two different acquisition systems used, and enable a more fair comparison between OECT and electrode recordings. The recordings were also digitally filtered with a 50Hz notch filter to remove line noise. See Supplementary Discussion for the influence of filtering on the background levels of the recordings. The calculation of the SNR was based on recordings filtered in this manner. The data were analysed using MATLAB (MathWorks). A Gabor wavelet time–frequency analysis was used to determine the frequency content of LFPs. CSD analysis of the simultaneously field potentials recorded with the penetrating probe was used to eliminate volume conduction and localize synaptic currents during epileptic discharges. CSD was computed as the second spatial derivative of the recorded raw LFPs (average of 44 events centred on the trough of the epileptic spikes on the deeper electrode of the penetrating probe). The 44 averaged signals superimposed to the CSD were digitally filtered with a 50-Hz notch filter. Power spectra of the recordings are shown in Supplementary Fig. S6 . Histology To assess the biocompatibility of parylene and PEDOT:PSS in the brain, we implanted a probe that consisted of an SU‐8 shank in the brain of a 500 g Long‐Evans rat. The shank was 5 mm long, had a width varying from 130 μm near the insertion tip to 400 μm at the end of the shank and a thickness of 50 μm. It was coated with a 2-μm thick conformal parylene film and, on one of its sides, with a PEDOT:PSS film. Parylene and PEDOT:PSS were deposited as described in the methods section. A 2 × 3 mm 2 craniotomy was performed in the right hemisphere above the somatosensory cortex, centred at the stereotaxic value of −3 in the antero‐posterior axis and −2 in the medio‐lateral axis, relative to Bregma. A single-shank silicon probe (Neuronexus A1 × 8–5 mm 50–177) was also implanted 1,000 μm apart in the same rat for comparison. Both probes were implanted to a final depth of 2 mm. After 30 days, the animal was killed and the probes removed from the brain. Tissue preparation and histological labelling were performed as described previously [39] . The rat was deeply anaesthetized with sodium pentobarbital injection (60 mg kg −1 , intraperitoneally) and perfused intracardially with a fixative solution containing 4% paraformaldehyde in 0.12 M sodium phosphate buffer (PB), pH 7.4. The rat received 300 ml of this fixative per 100 g of body weight. After perfusion, the brain was removed from the skull, post‐fixed in the same fixative for 1 h at room temperature and rinsed in 0.12 M PB for 1.5 h. It was then cryoprotected in a solution of 20% sucrose in 0.12M PB overnight at 4 °C, quickly frozen on dry ice and sectioned coronally at 40 μm on a cryostat. Sections were rinsed in 0.01 M PBS, pH 7.4, collected sequentially in tubes containing an ethylene glycol‐based cryoprotective solution and stored at −20 °C until histological processing. Every fifth section was stained with cresyl violet to determine the general histological characteristics of the tissue. How to cite this article: Khodagholy, D. et al . In vivo recordings of brain activity using organic transistors. Nat. Commun. 4:1575 doi: 10.1038/ncomms2573 (2013).